Electrical injection and detection of spin accumulation in silicon at 500 K with magnetic metal/silicon dioxide contacts The International Technology Roadmap for Semiconductors has identified the electron's spin angular momentum as a new state variable that should be explored as an alternative to the electron's charge for use beyond the size scaling of Moore's Law. A major obstacle has been achieving control of the spin variable at temperatures required for practical applications. Here we demonstrate electrical injection, detection and precession of spin accumulation in silicon, the cornerstone material of device technology, at temperatures that easily exceed these requirements. We observe Hanle precession of electron spin accumulation in silicon for a wide range of bias, show that the magnitude of the Hanle signal agrees well with theory, and that the spin lifetime varies with silicon carrier density. These results confirm spin accumulation in the silicon transport channel to 500 K rather than trapping in localized interface states, and enable utilization of the spin variable in practical device applications. The control of spin polarized carrier populations and currents offers a new paradigm for information processing in semiconductors [1] , [2] , [3] . Utilization of spin angular momentum as an alternate state variable provides additional functionality and performance for future electronic devices envisioned beyond the current roadmap [4] , [5] , [6] . Silicon (Si) is an ideal host for such a spin-based technology, because its low atomic mass and crystal inversion symmetry result in very small spin-orbit interactions and long spin lifetimes. Electrical generation, manipulation and detection of significant spin polarization in the semiconductor host at temperatures that meet commercial (85–100 °C) and military (125 °C) requirements are essential to this effort [7] . Electrical generation and detection of pure spin currents in Si using ferromagnetic (FM) metal/oxide tunnel barrier contacts have been demonstrated in lateral transport geometries for moderately doped Si ( n 007e2×10 18 cm −3 ) up to 125 K [8] , [9] , and to similar temperatures in metallic Si ( n ~5×10 19 cm −3 ) doped well above the metal–insulator transition (MIT) [10] . Recent work utilizing similar Al 2 O 3 tunnel barrier contacts on metallic Si ( n ~1×10 19 cm −3 ) reported spin-induced voltages attributed to spin accumulation in the Si directly under the injecting contact, which persisted up to 300 K, and exceeded theoretically expected values by two orders of magnitude [11] . Such large values of spin-induced voltages have been ascribed to spin trapping in localized interface states rather than the desired accumulation and transport in the semiconductor channel [12] . Here, we demonstrate electrical injection and detection of spin accumulation at temperatures up to 500 K in FM metal/silicon dioxide (SiO 2 )/ n -Si tunnel barrier structures in which the Si is both semiconducting and metallic in character, and present clear evidence that this spin accumulation occurs in the Si transport channel. SiO 2 has been a key element of the vast Si electronics industry, because this natural oxide is easy to form, and it produces an electrically stable self-interface with the low interface state density necessary for device operation. We observe Hanle precession of the electron spin accumulation in the Si channel under the FM metal/tunnel barrier contact for biases corresponding to both spin injection and extraction, and find that the magnitude of the Hanle signal decreases approximately linearly with temperature. In contrast with previous work, we provide clear evidence that the spin accumulation occurs in the Si channel rather than in localized interface states (a model suggested for Co/Al 2 O 3 /GaAs contacts [12] ) as follows: the measured spin resistance–area product is in good agreement with theory [12] , [13] , [14] ; and the spin lifetime clearly depends upon the Si carrier density, as expected from electron spin resonance work on bulk Si. These results demonstrate that spin accumulation in Si is viable as a basis for practical devices, which meet the operating temperatures specified for commercial (85 °C), industrial (100 °C) and military (125 °C) applications. Measuring spin accumulation Spin accumulation and precession directly under the magnetic tunnel barrier contact interface can be observed using a single contact for both spin injection and detection [11] , [12] , [15] . 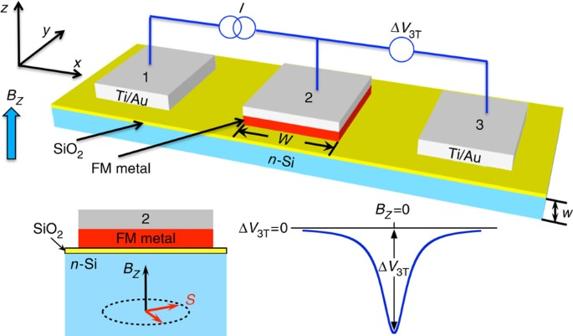Figure 1: Measurement geometry. In the three-terminal device measurement geometry, a current is applied to contacts 1 and 2, and a voltage is measured across contacts 2 and 3. Electrical spin injection produces spin accumulation in the transport channel under the magnetic contact 2 and a corresponding output voltage ΔV3T. When a magnetic fieldBzis applied, the injected spins precess and dephase, and ΔV3T(Bz) decreases to zero. The width of the magnetic contact isW=150 μm, and the thickness of the transport channel iswas indicated. This measurement configuration uses three terminals—two reference and one FM injector/detector, as shown in Figure 1 . The injection of spin polarized carriers produces a net spin accumulation described by the splitting of the spin-dependent electrochemical potential, Δ μ = μ up − μ down , which is detected as a voltage Δ V 3T = γ Δ μ /2 e , where γ ~0.4 is the tunnelling spin polarization of the FM tunnel contact (that is, the tunnel current has a spin polarization of 40%). When a magnetic field B z is applied perpendicular to the electron spin direction (sample surface), the spins precess at the Larmor frequency ω L = gμ B B z / [hmacr] , resulting in a reduction of the net spin accumulation to zero due to precessional dephasing (Hanle effect) [16] . Here, g is the Lande g -factor ( g= 2 for Si), μ B the Bohr magneton and [hmacr] is the reduced Planck's constant. The magnitude of the voltage Δ V 3T ( B z ) decreases with B z with an approximately Lorentzian line shape given by Δ V 3T ( B z )=Δ V 3T (0)/[1+( ω L τ s ) 2 ], and the spin lifetime τ s is obtained from fits to this line shape. In contrast with four-terminal non-local measurements [9] , [10] , [17] , three-terminal measurements enable one to focus on and probe the characteristics of the spin system in the semiconductor directly beneath the spin-injecting contact. As the magnetic contact interface is likely to introduce additional scattering and spin relaxation mechanisms not present in the bulk, the region of the semiconductor directly beneath the contact is expected to be a critical factor in any future spin technology. Figure 1: Measurement geometry. In the three-terminal device measurement geometry, a current is applied to contacts 1 and 2, and a voltage is measured across contacts 2 and 3. Electrical spin injection produces spin accumulation in the transport channel under the magnetic contact 2 and a corresponding output voltage Δ V 3T . When a magnetic field B z is applied, the injected spins precess and dephase, and Δ V 3T ( B z ) decreases to zero. The width of the magnetic contact is W= 150 μm, and the thickness of the transport channel is w as indicated. Full size image Hanle spin precession data The Si samples are n -doped just above and below the MIT (~5×10 18 cm −3 ). Samples with four different carrier densities were studied, and multiple devices were measured on each sample. Data from two samples are typically presented (sample A: 3×10 19 cm −3 and sample B: 3×10 18 cm −3 ). 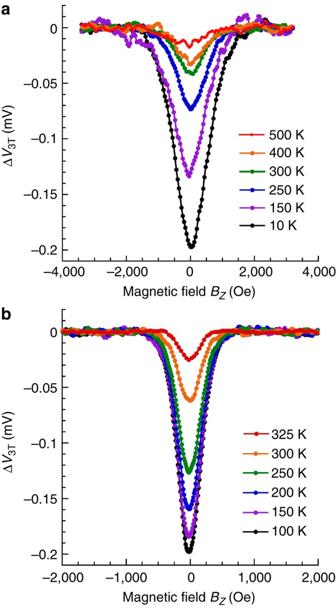Figure 2: Hanle effect data. Three-terminal Hanle curves for temperatures indicated for (a) sample A,I=−500 μA, and (b) sample B,I=−7 μA (both spin injection). Spin precession is clearly visible to 500 K for sample A. The maximum bias voltage used wasV=−1 V. The higher resistance of sample B prevented larger bias currents within the 1 V bias limit. Control devices with non-magnetic contacts show no Hanle effect. Note the scale change on thexaxis. Hanle curves obtained at temperatures of 10–500 K are shown in Figure 2a,b for a fixed bias current I =−500 and −7 μA for sample A and B, respectively. For negative bias, spin-polarized electrons with net majority spin are injected from the FM into the Si [18] . A maximum bias voltage of 1 V was used for all devices, and a quadratic background has been subtracted from the data. As B z increases, precessional dephasing reduces the spin accumulation and Δ V 3T ( B z ) decreases to zero. Spin precession as manifested by the Hanle signal is clearly observed to 500 K, the maximum temperature accessible in our measurement system. Figure 2: Hanle effect data. Three-terminal Hanle curves for temperatures indicated for ( a ) sample A, I =−500 μA, and ( b ) sample B, I =−7 μA (both spin injection). Spin precession is clearly visible to 500 K for sample A. The maximum bias voltage used was V =−1 V. The higher resistance of sample B prevented larger bias currents within the 1 V bias limit. Control devices with non-magnetic contacts show no Hanle effect. Note the scale change on the x axis. Full size image Comparison of Hanle signal amplitude with theory The amplitude of the Hanle signal agrees well with that expected from the theory of spin injection into a semiconductor channel in the diffusive regime [13] , [14] , indicating that spin accumulation occurs in the semiconductor channel rather than in localized interface states. The amplitude of the Hanle signal at 300 K for sample A, Δ V 3T ( B z =0)~0.04 meV, corresponds to a spin resistance R s =Δ V 3T ( B z =0)/ I ~0.08 Ω, or equivalently a spin resistance–area product R s · A ~1,200 Ω μm 2 for the 150×100 μm 2 contact. The value at 10 K is R s · A ~6,000 Ω μm 2 . These are in excellent agreement with the value predicted by theory [12] , [13] , [14] as given by r 1 =( ρL SD )( W/w )~3,000 Ω μm 2 using parameters measured for our sample. Here, ρ is the Si resistivity, L SD is the spin diffusion length obtained from the Hanle line shape as described below, W is the contact width, w is the semiconductor channel thickness, and we assume that the active channel thickness over which spin accumulation occurs in very thick samples is limited by the spin diffusion length. The corresponding values for sample B at 300 K are R s · A ~129 kΩ μm 2 and r 1 ~15 kΩ μm 2 . The poorer agreement with theory is attributed to the fact that sample B is non-metallic in character, with a significant depletion width ~15–20 nm, and the accompanying band bending in the Si is not included in the theory. For comparison, Tran et al . [12] found that their measured R s · A value for Co/Al 2 O 3 /GaAs three-terminal devices was over three orders of magnitude larger than that predicted by theory, leading them to conclude that spin accumulation occurred in highly localized interface states rather than in the semiconductor itself. Dash et al . [11] also found that their measured values for NiFe/Al 2 O 3 /Si ( n ~2×10 19 cm −3 ) three-terminal devices were about two orders of magnitude larger than that predicted by theory. Both of these studies used Al 2 O 3 as the tunnel barrier, a material known to produce relatively high densities of interface states on either GaAs or Si [19] . The fact that our measured values are in good agreement with the theory (which assumes zero interface spin accumulation) is consistent with the lower interface state density of the SiO 2 /Si system, and provides the first of two pieces of evidence that spin accumulation occurs in the Si itself rather than in localized interface states. Spin lifetimes The line shape of the three-terminal Hanle data can be fit to obtain a value for the spin lifetime τ s by using an expression analogous to the classic optical Hanle effect, that is, a simple Lorentzian given by Δ V 3T ( B z )=Δ V 3T (0)/[1+( ω L τ s ) 2 ] [16] . This procedure has been shown to give a lower bound for τ s [11] . 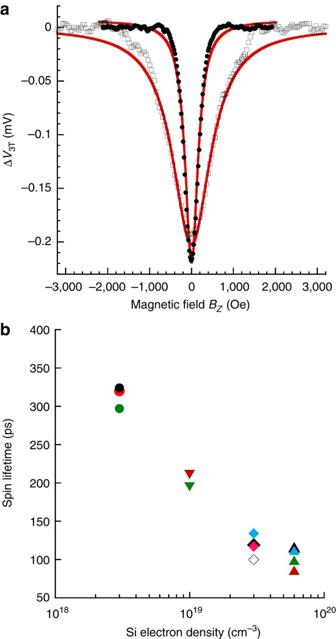Figure 3: Dependence of spin lifetime on electron density. (a) Hanle curves taken in the three-terminal geometry at 10 K for sample A (open symbols,n=3×1019cm−3, I=−500 μA) and sample B (closed symbols,n=3×1018cm−3,I=−7 μA). The solid lines are Lorentizian fits to the Hanle data and yield spin lifetimesτs=100 and 320 ps for sample A and B, respectively. (b) Spin lifetime as a function of the Si carrier concentration at 10 K. Each coloured data point represents a separate device on which many Hanle measurements were made, and the error bar for each is ±10 ps. The symbols distinguish the FM metal used: solid symbols correspond to devices with Ni0.8Fe0.2contacts, whereas open symbols correspond to Co0.9Fe0.1contacts. A bias voltage ~0.9 V was used for all data shown. Typical Lorentzian fits are shown in Figure 3a for both samples, and yield spin lifetimes of 100±10 and 320±10 ps for sample A (3×10 19 cm −3 ) and B (3×10 18 cm −3 ), respectively, at 10 K. The dependence of τ s on the Si electron density is shown in Figure 3b . Each data point plotted represents a separate device on which many measurements were made. The decrease in τ s with increasing carrier concentration is consistent with the electron spin resonance (ESR) results for bulk Si, and attributed to impurity-dominated Elliot–Yafet spin relaxation processes [20] , [21] , [22] , [23] . The fact that the spin lifetime exhibits a clear dependence upon the Si carrier density consistent with the trend observed in bulk Si [20] , [22] , [23] provides further evidence that the spin accumulation/precession indeed occurs in the Si channel rather than in localized interface states. Figure 3: Dependence of spin lifetime on electron density. ( a ) Hanle curves taken in the three-terminal geometry at 10 K for sample A (open symbols, n =3×10 19 cm −3 , I=−500 μA) and sample B (closed symbols, n =3×10 18 cm −3 , I =−7 μA). The solid lines are Lorentizian fits to the Hanle data and yield spin lifetimes τ s =100 and 320 ps for sample A and B, respectively. ( b ) Spin lifetime as a function of the Si carrier concentration at 10 K. Each coloured data point represents a separate device on which many Hanle measurements were made, and the error bar for each is ±10 ps. The symbols distinguish the FM metal used: solid symbols correspond to devices with Ni 0.8 Fe 0.2 contacts, whereas open symbols correspond to Co 0.9 Fe 0.1 contacts. A bias voltage ~0.9 V was used for all data shown. Full size image These spin lifetime values are about an order of magnitude smaller than those obtained by ESR for corresponding doping levels in bulk Si [22] , [24] . This may be a consequence of the lower bound for τ s produced by the Lorentzian fitting procedure [11] , but is also a trend that we have observed previously and attributed to the vicinity of the contact interface [17] , where both the reduced symmetry and surface/impurity scattering are likely to produce more rapid spin relaxation than in the bulk. The spin lifetime shows little variation with temperature, and similar values are obtained at 300 K. Ochiai and Matsuura [22] also found τ s to exhibit a weak temperature dependence in bulk Si ( n =3.4×10 19 cm −3 (As)), which they attributed to the metallic character of the sample, where impurity-dominated spin-orbit interaction dominates spin relaxation for a wide temperature range. The proximity of the tunnel barrier interface is also expected to contribute by introducing relaxation mechanisms not present in the bulk. First, the reduced symmetry and increased scattering noted above may obscure other temperature-dependent effects. Second, spins can readily diffuse between the Si and FM metal contact through the relatively transparent tunnel barrier necessary for reasonable spin current flow (>1 μA)—as the spin lifetime is insensitive to temperature in the FM, this masks any dependence one might expect to see in the Si. The spin lifetimes thus extracted in the three-terminal geometry reflect the environment in close proximity to the contact. Spin diffusion lengths and temperature dependence The spin diffusion length is given by L SD =( Dτ s ) 1/2 , where D is the diffusion constant calculated from the measured carrier concentration and mobility. 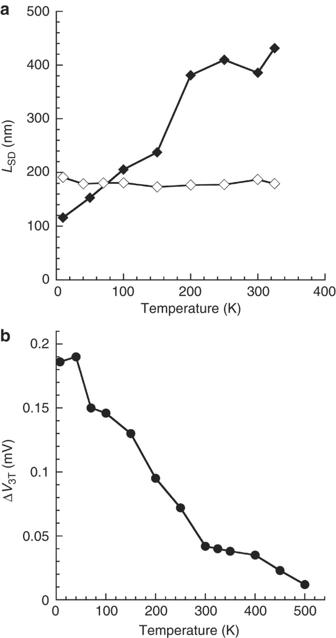Figure 4: Temperature dependence. (a) Spin diffusion lengthLSDas a function of temperature for sample A (open symbols,n=3×1019cm−3) and sample B (closed symbols,n=3×1018cm−3). (b) Plot of the magnitude of three-terminal voltage as a function of temperature for sample A. We obtain L SD ~190 nm (120 nm) for sample A (B) at 10 K. The temperature dependence of the spin diffusion length is summarized in Figure 4a . For sample A, L SD exhibits little variation with temperature, because neither D nor τ s does. As noted previously, Ochiai and Matsuura [22] also found τ s to exhibit a weak temperature dependence in heavily doped bulk Si. For sample B, L SD increases with temperature, a trend due largely to the temperature dependence of D=μkT/q for a non-degenerate system, where μ is the mobility. L SD reaches a value ~400 nm near room temperature and above, demonstrating that practical devices based on spin transport in Si are viable with conventional lithographic and fabrication techniques found in most Si fabrication lines. These spin diffusion lengths are shorter than those measured previously in Si epilayers using a four-terminal non-local geometry (~1 μm for n =3×10 18 cm −3 at 10 K) [9] , [17] . In the four-terminal geometry, the spin diffuses laterally away from the contact and samples non-contact regions of the Si before detection, so that the spin properties extracted represent some weighted average of those for the non-contact and contact regions. In contrast, the three-terminal geometry probes the Si directly at the contact interface, where additional spin scattering mechanisms are likely to be present, as discussed in the previous paragraph. Figure 4: Temperature dependence. ( a ) Spin diffusion length L SD as a function of temperature for sample A (open symbols, n =3×10 19 cm −3 ) and sample B (closed symbols, n =3×10 18 cm −3 ). ( b ) Plot of the magnitude of three-terminal voltage as a function of temperature for sample A. Full size image The temperature dependence of the Hanle amplitude is shown in Figure 4b . The amplitude of the signal Δ V 3T ( B z =0) decreases monotonically with temperature, a trend inconsistent with that of the spin diffusion length and lifetime, indicating that other factors, such as spin injection/detection efficiency, may be responsible. The detector efficiency, for example, has been shown to exhibit pronounced bias dependence at a fixed temperature [25] . The temperature dependence of the detection efficiency has not been addressed to date, and is beyond the scope of this paper. Bias dependence of Hanle signal Spin accumulation can also be generated by reversing the bias so that electrons flow from Si into the FM metal, referred to as spin extraction [17] , [26] . In this case, minority spin polarization builds in the Si because of preferential transmission of majority spin electrons into the FM tunnel contact, and the Hanle curve Δ V 3T ( B z ) (proportional to Δ μ ) is expected to change the sign. 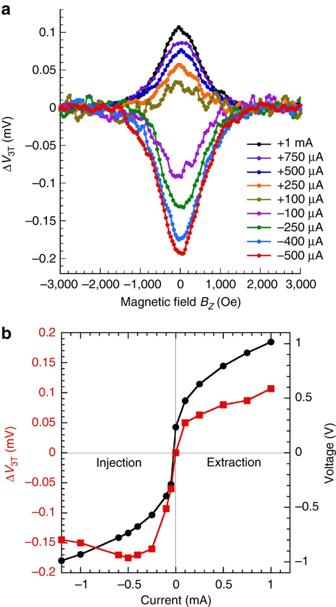Figure 5: Bias dependence. (a) Three-terminal Hanle curves for different values of the injection current atT=10 K for sample A. Negative bias indicates injection of majority spin electrons from the FM contact into the Si. Positive bias indicates the extraction of majority spin from Si into FM contact, which leaves an accumulation of minority spin in Si, consistent with the sign reversal of the measured voltage. (b) Plot of the magnitude of three-terminal voltage ΔV3Tas a function of injection current (red squares), and theI–Vcharacteristic of the FM tunnel barrier contact (black circles). The lines are guides to the eye. This is confirmed by the series of Hanle curves shown in Figure 5a for sample A, where the bias voltage applied to the tunnel barrier contact is varied from negative (injection) to positive (extraction), with a corresponding inversion of the Hanle signal. Figure 5: Bias dependence. ( a ) Three-terminal Hanle curves for different values of the injection current at T =10 K for sample A. Negative bias indicates injection of majority spin electrons from the FM contact into the Si. Positive bias indicates the extraction of majority spin from Si into FM contact, which leaves an accumulation of minority spin in Si, consistent with the sign reversal of the measured voltage. ( b ) Plot of the magnitude of three-terminal voltage ΔV 3T as a function of injection current (red squares), and the I–V characteristic of the FM tunnel barrier contact (black circles). The lines are guides to the eye. Full size image The bias dependence of the three-terminal voltage Δ V 3T ( B z =0) is summarized in Figure 5b together with the I–V plot of the magnetic tunnel barrier contact. Δ V 3T is linear for low biases (±100 μA), but exhibits pronounced asymmetry at higher bias. For large positive bias (extraction), the behaviour is consistent with the I–V characteristic of the contact, that is, the spin accumulation monotonically increases, roughly tracking the injected current density, as one might expect. However, at negative bias (injection), Δ V 3T ( B z =0) achieves a larger absolute magnitude indicating higher spin accumulation, but then saturates and slightly decreases. This is not fully understood at present, but may be because of either a bias dependence of the detector efficiency [25] or a spin bottleneck effect [27] —majority spin electrons flowing from the FM contact to the Si see a spin resistance generated by spin accumulation in the Si within a spin diffusion length of the contact interface, whereas unpolarized electrons flowing from the Si will not experience this effect. Note that a larger spin accumulation per unit current density is generated for injection than for extraction. Control experiments Control experiments were performed to evaluate and exclude contributions from several potential spurious effects. Devices fabricated with non-magnetic contacts show no Hanle effect and negligible magnetic field dependence. The magnetoresistance effect in Si (due to Lorentz deflection of electrons by the magnetic field) is found to be negligible in our samples. The anisotropic magnetoresistance in the FM metal contact produced by rotation of the magnetization out of plane due to the applied field B z is found to be at most 2% of the measured Hanle signal, significantly smaller than the Hanle curves shown here. The physical location within the sample structure of the spin accumulation giving rise to the Hanle signal in the three-terminal geometry is a matter of current debate, and such data require careful interpretation. One would reasonably expect spin injection from a FM contact to result in spin accumulation in the semiconductor channel. This was the basis for the original theory of spin injection in the diffusive regime applied at a single ferromagnet/semiconductor interface, which predicted a spin resistance of r 1 =( ρL SD )( W/w ) in units Ω μm 2 [13] , [14] . However, recent experimental work has shown that spin accumulation can occur instead in localized interface states, giving rise to a much larger signal Δ V 3T ( B z =0) than expected [12] , typically expressed as the spin resistance–area product R s · A =Δ V 3T ( B z =0)· A / I . This interface state model was developed by Tran et al . [12] to describe three-terminal Hanle measurements on Co/Al 2 O 3 /GaAs samples. Because their Hanle signal was 10 3 times larger than that predicted by theory, they concluded that spin accumulation developed in localized states with long spin lifetimes near the tunnel barrier/semiconductor interface, rather than in the GaAs channel. Effectively, in the expression for r 1 , w decreases by ~10 2 –10 3 to a value w ~1 nm commensurate with an effective interface width. Thus, in cases where the measured Hanle signal R s · A ≫ r 1 , spin injection/transport in the semiconductor itself is not necessarily indicated. The oxide/GaAs interface is well known to have a high density of interface states, which has thwarted development of a metal–oxide–semiconductor transistor technology [19] . Similarly, Al 2 O 3 /Si interfaces formed by sputter or electron beam deposition of the oxide exhibit large interface state densities [28] , which may contribute to the large Hanle signals recently measured for NiFe/Al 2 O 3 /Si three-terminal devices [11] —these values were about two orders of magnitude larger than that predicted by theory. In contrast, the R s · A values presented here for the FM/SiO 2 /Si three-terminal devices are in very good agreement with the original theory over a wide temperature range. In addition, the spin lifetimes show a clear correlation with the Si carrier density consistent with ESR data for bulk Si. These data lead us to rule out spin accumulation in interface states, and conclude that our results demonstrate spin injection, accumulation and precession in the n -doped Si channel at temperatures up to 500 K. Non-local four-terminal Hanle measurements also provide clear indication of spin transport in the Si channel, although to date such data extend only to T~125 K [9] , [10] , [17] , [29] . In summary, we have observed Hanle precession of the electron spin in Si at temperatures up to 500 K, demonstrating electrical spin injection/detection with FM metal/SiO 2 tunnel barrier contacts. We find that the magnitude of the Hanle signal is in good agreement with theory, and decreases approximately linearly with temperature over the range 10–500 K. Lorentzian fits to the Hanle curves yield spin lifetimes of ~320 (100) ps and spin diffusion lengths of ~120 (190) nm at 10 K for the lower (higher) n -doping levels at a bias voltage ~0.9 V. These values are insensitive to temperature for carrier densities in the metallic regime, that is, above the MIT. Our results demonstrate that the spin accumulation in Si is viable as a basis for practical devices, which meet the operating temperatures specified for commercial (85 °C), industrial (100 °C) and military (125 °C) applications. Additional challenges remain before a practical technology can be realized, and some solutions have already been outlined. Behin–Aein et al . have argued that it may be inefficient and unnecessary to convert the spin accumulation in the semiconductor to a conventional measure such as an output voltage [6] . They argue that such repeated spin-to-charge conversion wastes energy and negates the advantage of a spin state variable, and propose instead a logic/memory device that uses spin at every stage of its operation using nanomagnets as digital spin capacitors to store information. Spin gain has also been identified as a challenge, with preliminary experiments pointing towards a solution, albeit at low temperatures [30] . Several manifestations of a transistor exhibiting spin gain have been proposed and modelled, including the Si-based spin-MOSFET [31] , and a transistor, which incorporates a magnetic semiconductor as the base [32] . We hope that our results presented here enable a practical realization of a spin-based semiconductor device technology. Sample properties Samples with four different carrier densities were studied, ranging 3×10 18 –6×10 19 cm −3 as determined by Hall measurements at room temperature. Samples were fabricated on two types of n -doped Si(001) substrates. Sample A was a Si-on-insulator wafer with a 2-μm-thick active Si layer, n =3×10 19 cm −3 (As) and a resistivity of 2 mΩ cm at room temperature. The resistivity showed little change with decreasing temperature, confirming the metallic behaviour. Sample B was a 350-μm-thick prime wafer with n =3×10 18 cm −3 (Sb) and a resistivity of 10 mΩ cm at 300 K, which increased with decreasing temperature, indicating the semiconducting behaviour. The other two samples were both Si-on-insulator wafers with carrier densities of 1×10 19 and 6×10 19 cm −3 . Sample processing and fabrication Each sample was first etched with 5% hydrofluoric acid and rinsed with deionized water to remove the native oxide and produce a hydrogen-terminated surface, and then introduced into a sputtering system with a base pressure in the high 10 −8 Torr range. The plasma is initiated with a 50 mTorr mixture of 1:1 Ar+O 2 (at a flow rate of 15 standard cubic centimeters per minute (SCCM) each) and a radio frequency (RF) plasma power of 50 W. After changing to an O 2 only atmosphere of 100 mTorr (at a flow rate of 30 SCCM) and increasing the plasma power to 120–140 W, the sample is then moved to the vicinity of the plasma, where the SiO 2 tunnel barrier is formed by oxidizing the surface in this oxygen plasma at room temperature for 10 min. A range of 15–25 nm of either Co 0.9 Fe 0.1 or Ni 0.8 Fe 0.2 was then sputter deposited in situ on the SiO 2 using a magnetron sputtering source with a pulsed direct current power supplied and operated at 100 W at a rate of 10 nm min −1 at the same temperature. Conventional photolithography and wet chemical etching were used to produce contact layouts as those shown in Figure 1 . The 150×100 μm magnetic metal contact is capped with 10 nm Ti/100 nm Au, which was also used for the two ohmic reference contacts, and bond pads for the electrical connections are electrically isolated from the Si using 100 nm of Si 3 N 4 . Characterization of tunnel barriers The integrity of the SiO 2 tunnel barrier was confirmed by using typical I–V analysis procedures [33] , including successful fits of the I–V curves with the Brinkman–Dynes–Rowell model, and measuring the temperature dependence of the zero bias resistance. 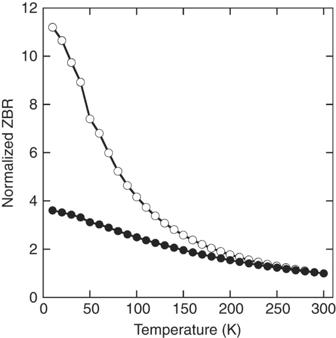Figure 6: Tunnel barrier characterization. Normalized zero bias resistance (zbr) as a function of temperature measured for the SiO2tunnel barriers utilized, showing a weak temperature dependence characteristic of tunnelling. The two curves show the range of behaviour exhibited by devices fabricated in different processing runs. The normalized zero bias resistance of the tunnel barrier contact, defined as R(T)/R(300 K), exhibited modest temperature dependence as shown in Figure 6 , which has been argued to be a more rigorous and reliable indicator of a pinhole free tunnel barrier than simple application of the usual Rowell criteria [34] . Figure 6: Tunnel barrier characterization. Normalized zero bias resistance (zbr) as a function of temperature measured for the SiO 2 tunnel barriers utilized, showing a weak temperature dependence characteristic of tunnelling. The two curves show the range of behaviour exhibited by devices fabricated in different processing runs. Full size image Diffusion constant The diffusion constant D is calculated from the measured carrier concentration and mobility using either the Einstein relation D = μkT/q for non-degenerate systems, or the full Fermi–Dirac expansion D =(2 μ kT / q )( F 1/2 ( η F )/ F −1/2 ( η F ) for degenerate systems (that is, when E F moves into the conduction band), where F 1/2 ( η F ) and F −1/2 ( η F ) are the Fermi–Dirac integrals of order ½ and −½, respectively, and η F ≡( E F − E C / kT ) [33] . How to cite this article: Li, C. H. et al . Electrical injection and detection of spin accumulation in silicon at 500 K with magnetic metal/silicon dioxide contacts. Nat. Commun. 2:245 doi: 10.1038/ncomms1256 (2011).